Massive band gap variation in layered oxides through cation ordering The electronic band gap is a fundamental material parameter requiring control for light harvesting, conversion and transport technologies, including photovoltaics, lasers and sensors. Although traditional methods to tune band gaps rely on chemical alloying, quantum size effects, lattice mismatch or superlattice formation, the spectral variation is often limited to <1 eV, unless marked changes to composition or structure occur. Here we report large band gap changes of up to 200% or ~2 eV without modifying chemical composition or use of epitaxial strain in the LaSrAlO 4 Ruddlesden-Popper oxide. First-principles calculations show that ordering electrically charged [LaO] 1+ and neutral [SrO] 0 monoxide planes imposes internal electric fields in the layered oxides. These fields drive local atomic displacements and bond distortions that control the energy levels at the valence and conduction band edges, providing a path towards electronic structure engineering in complex oxides. In superlattices and heterostructures, the Coulombic interaction between adjacent atomic layers of (nominally) charged and/or neutral planes can create internal electric fields [1] , [2] , [3] that induce or alter many functional electronic, ferroic and optical properties [4] , [5] , [6] , [7] , [8] , [9] . In the majority of atomically layered oxides explored to date, however, the heterostructures are constructed by interleaving two or more bulk materials, often perovskite ‘blocks’ with well-defined three-dimensional connectivity [10] , [11] , [12] , [13] , [14] , [15] . Rarely are the starting oxides natural heterostructures themselves, for example, Aurivillius, Dion-Jacobson or the Ruddlesden-Popper (RP) phases. The latter (ABO 3 ) n /(AO) (also denoted as A n +1 B n O 3 n +1 ) RP structure has n ABO 3 perovskite blocks stacked along the [001] direction with an extra sheet of AO rock-salt layers interleaved every n perovskite layers. This geometry disconnects the BO 6 octahedra along one direction and imposes severe constraints on the nearest-neighbour interactions [16] , promoting anisotropy in the structure-derived electronic, transport and magnetic properties, which contrasts sharply with the 3D perovskite analogues [17] , [18] , [19] , [20] . Indeed, the RP structure dimensionality [21] , [22] , that is, systematic stacking of the n layers along [001] direction, has recently been exploited [23] in combination with epitaxial strain to achieve highly tunable low-loss dielectrics. Yet, the range over which band gap control may be achieved in oxide heterostructures derived from two-dimensional building blocks remains less explored and largely unknown. In n =1 RP oxides, there are three types of A-cation arrangements that produce [001]-cation ordering without changing the number of formula units per cell relative to the A 2 BO 4 aristotype [24] . We denote the stoichiometry of the ordered variants as AA′BO 4 , where A and A′ are two chemically distinct cations with 100% site occupancy. In the context of this work, A, A′ and B are La 3+ , Sr 2+ and Al 3+ cations, respectively, and the corresponding n =1 RP oxide stoichiometry is denoted as LaSrAlO 4 . The A-cation ordering scheme produces the long-range periodic ordering of [LaO] 1+ and [SrO] 0 planes in the crystal structure as shown in Fig. 1 . Normally, such long-range chemical orderings are experimentally detected using diffraction measurements through the appearance of superlattice reflections, which are forbidden in a fully disordered or solid solution phase. As there are three different ways to order [LaO] 1+ and [SrO] 0 planes without cell multiplication, we introduce two structural parameters, λ and ξ , that provide a measure for classifying the orderings, which have both the same composition and number of formula units. This scheme can also describe longer period sequences not directly examined herein, and is also useful to describe the interlayer interactions across disconnected BO 6 units [25] . λ and ξ capture the relative proximities of the positively charged [LaO] 1+ and neutral [SrO] 0 monoxide layers along [001] direction (see Fig. 1 ). λ defines the separation, quantified in terms of the number of metal oxide planes along [001] direction, between two chemically equivalent [LaO] 1+ (or [SrO] 0 ) layers, and ξ defines the separation between two nearest chemically inequivalent [LaO] 1+ and [SrO] 0 layers with distinct charged states. 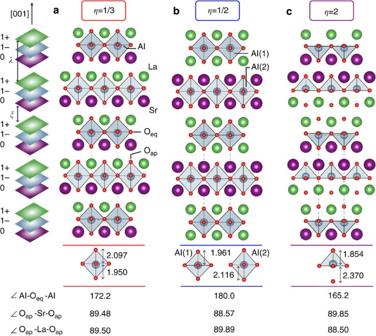Figure 1: Equilibrium LaSrAlO4crystal structures. DFT-PBEsol ground states for the three cation ordered configurations (a)η=1/3, (b)η=1/2 and (c)η=2, whereη=ξ/λ.ξ(distance between two nearest chemically inequivalent [LaO]1+and [SrO]0layers) andλ(distance between two chemically equivalent [LaO]1+(or [SrO]0) layers) are defined in the schematic of charged atomic AO and BO2layers that corresponds to the atomic arrangement in (a). Note that for theη=1/3 arrangement in (a), there are two ways to defineξas described in ref.25. Here we takeξto be the minimum value, because the interactions from the nearest-neighbour monoxide layers are unscreened by an interleaved perovskite block. Theη=1/2 configuration shown in (b) has two crystallographically inequivalent Al sites. In (c) the coordination of Al is reduced to fivefold square pyramidal. Colour coding and naming scheme based on the local atomic structure in parentheses: (a) red box (polar), (b) blue box (non-polar) and (c) purple box (anti-polar). Bond lengths and angles are given in units of angstroms and degrees, respectively. Figure 1: Equilibrium LaSrAlO 4 crystal structures. DFT-PBEsol ground states for the three cation ordered configurations ( a ) η =1/3, ( b ) η =1/2 and ( c ) η =2, where η = ξ / λ . ξ (distance between two nearest chemically inequivalent [LaO] 1+ and [SrO] 0 layers) and λ (distance between two chemically equivalent [LaO] 1+ (or [SrO] 0 ) layers) are defined in the schematic of charged atomic AO and BO 2 layers that corresponds to the atomic arrangement in ( a ). Note that for the η =1/3 arrangement in ( a ), there are two ways to define ξ as described in ref. 25 . Here we take ξ to be the minimum value, because the interactions from the nearest-neighbour monoxide layers are unscreened by an interleaved perovskite block. The η =1/2 configuration shown in ( b ) has two crystallographically inequivalent Al sites. In ( c ) the coordination of Al is reduced to fivefold square pyramidal. Colour coding and naming scheme based on the local atomic structure in parentheses: ( a ) red box (polar), ( b ) blue box (non-polar) and ( c ) purple box (anti-polar). Bond lengths and angles are given in units of angstroms and degrees, respectively. Full size image It is the delicate balance of electrostatic interactions among these layers that provides a handle to direct the Al–O bond distortions and ionicity in LaSrAlO 4 through A-site ordering. The ratio of these parameters, η = ξ / λ , is used to distinguish each phase by layer sequence; a local structural description of how η distinguishes each variant is described below and emphasized by the colour-coding scheme in Fig. 1 . Here, we seek to understand the effects of λ and ξ on the electronic band gap in LaSrAlO 4 and predict its change on ordering. Experiments of the solid solution phase ( η =0) report an indirect band gap ( E g ) near ~4–5 eV (refs 26 , 27 , 28 ), whereas the proposed A-site ordered structures examined herein remain to be synthesized and are unknown. More recently, we computationally demonstrated the importance of A-site cation ordering and η parameter on the rock-salt layers of n =1 RPs in metallic LaANiO 4 with correlated electrons, where A=Ca 2+ , Sr 2+ and Ba 2+ (ref. 25 ). The ordering sequence of A-site cations on (001) AO monoxide planes in LaANiO 4 RP oxides alters the electrostatic interactions, through a so-called ‘electrostatic chemical strain’ (ECS) effect [25] , and was used to manipulate the 3 d -orbital structure at the Fermi level. It is termed an ECS effect, because of the manner in which these artificial oxides are constructed. The unit cell is obtained by ordering nominally positively charged [LaO] 1+ and neutral [AO] 0+ metal oxides, thereby creating a continuously varying ‘electrostatic’ potential due to dipolar interactions derived from [LaO] 1+ and [AO] 0+ ordering not appearing in the solid solution material. Our density functional theory (DFT) calculations revealed that the bond stresses [29] from the chemically imposed local electric fields are accommodated by changes to the bond lengths and bond angles. It is the change in bond length between an ordered and disordered (solid solution) system relative to the disordered system that leads to the local microscopic ‘strain’ within the ECS framework. Furthermore, the charge state of the ions and their relative sizes, which we refer to as chemistry of the element, were also identified to be important. Thus, the interplay of electrostatics, bond strain and chemistry manifests as an ECS in layered oxides with ordered cation sublattice. In this work, we focus on a prototypical insulating RP oxide, LaSrAlO 4 , and show that A-cation ordering, without any change to stoichiometry, enables deterministic control over the electronic band gap of the material ( E g ). We report that the arrangement of the AO monoxide [LaO] 1+ and [SrO] 0 layers within a single-unit cell directs the magnitude of E g through internal electric fields, which drive bond distortions producing large reductions in the conduction band minimum: it varies by ~2 eV in magnitude over the monoxide layering sequences explored. Our work establishes heterovalent A-cation ordering as a novel ‘control knob’ in addition to epitaxial strain and layer dimensionality ( n ) to design the properties of artificial complex oxides from modular building blocks that are naturally layered. Energetics We obtain equilibrium LaSrAlO 4 cation ordered structures by systematically exploring the energetics of various lattice modes obtained from computed phonon dispersion curves for each sequence. Our frozen phonon calculations indicate the high symmetry structures of all three LaSrAlO 4 sequences are dynamically stable (see Supplementary Figs 1–3 ). Figure 1 depicts the ground state structures for the three A-site ordered variants. No AlO 6 octahedral tilting or rotations occur, only bond elongations and rumpling distortions, that is, the Al and O atoms are displaced away from the Al-O equatorial plane. On comparing the total energies for the three sequences, the η =2 sequence is found to be the most stable ordered variant ( Fig. 1c ), with the η =1/3 and 1/2 sequences 4 and 242 meV per formula unit (f.u. ), respectively, higher in energy (see Supplementary Fig. 4 ). Ground-state structures and dynamical charges The ground-state structure for the η =1/3 sequence is polar (space group I 4 mm , Fig. 1a ) owing to the A-cation compositional order removing inversion symmetry [24] . The lattice tetragonality ( c / a ) is 3.324, and the AlO 6 octahedra have four crystallographically equivalent equatorial (eq) Al–O eq and two unique (one short and one long) apical (ap) Al–O ap bonds, which give rise to an electric polarization of 7.2 μC cm −2 along the [001] direction as obtained from the Berry phase method. The asymmetry in the Al–O ap bond lengths arises from the negatively charged [AlO 2 ] 1− layer being interleaved between a positively charged [LaO] 1+ and a neutral [SrO] 0 layer. The O eq atoms in the [AlO 2 ] 1− layer are attracted towards the positively charged [LaO] 1+ layer, which simultaneously buckles the O eq –Al–O eq bonds so they deviate from 180°. Interestingly, we find no anomalously large or small Born effective-charges Z * (relative to the nominal charge) in the ground state ( Table 1 ); however, anisotropy between the in-plane ( and ) and out-of-plane is evident. Table 1 Summary of the Born effective-charge tensors. Full size table In contrast, the η =1/2 LaSrAlO 4 structure is centrosymmetric and non-polar (space group P 4/ mmm ). Figure 1b shows that, although the AO monoxide sequence splits the Al sites into two distinct AlO 2 sublattices, we find that the c / a value (3.318) is close to that of η =1/3. Unlike the η =1/3 sequence, where the O eq –Al–O eq bond angles are <180 ° and there are two Al–O ap bonds, here there is no rumpling ( ∠ O eq –Al–O eq =180°). At each site, the two Al–O ap bonds are also of equal length; however, the relative lengths of the Al–O ap bonds differ between the two AlO 6 octahedra. In the [LaO|Al(1)O 2 |LaO] and [SrO|Al(2)O 2 |SrO] perovskite-like blocks, the Al–O ap bonds are 1.96 and 2.12 Å, respectively, indicating a markedly different coordination and chemical environment owing to the cation order ( Fig. 1b ). Indeed, while the in-plane (and ) for both Al sites is close to the nominal ionic charge of +3 e , the out-of-plane components show significant deviations from the nominal value that depend on the adjacent monoxide layer chemistry. The values are 2.57 e and 3.70 e for Al(1) and Al(2), respectively, with the shorter Al–O ap bond lengths reflecting stronger covalent interactions [30] with the O(2) ap atoms in the LaO layer. Note that the sign of the charge anisotropy Δ Z (La) also changes from negative (in η =1/3) to a positive value in this non-polar variant, indicating that [LaO] 1+ layers are more sensitive to cation ordering relative to the [SrO] 0 layers (despite ξ being the same as before). Similar to the η =1/3 phase, for the η =2 aluminate there are [AlO 2 ] 1− layers interleaved between [LaO] 1+ and [SrO] 0 , yet the structure is centrosymmetric ( P 4/ mmm ) due to anti-polar displacements rather than symmetric stretching. The O eq atoms shift towards the [LaO] 1+ layers and a significant disproportionation of the Al–O ap bonds occurs with large deviations of the O eq –Al–O eq bond angles away from 180°. The electrostatic effects within the unit cell are further enhanced, because the two [LaO] 1+ layers are in close proximity to one another, which leads to a repulsive interaction. The [LaO] 1+ –[LaO] 1+ repulsion is evident in the asymmetry of the Al–O ap bond lengths, where we find 2.37 and 1.85 Å for the O ap oxygen in the [LaO] 1+ and [SrO] 0 layers, respectively. The overall consequence of the enhanced electrostatic effects are that the η =2 LaSrAlO 4 structure has the largest c / a axial ratio (3.44), compared with other ordered variants, including the random alloy (3.36) [31] . Except for a large for the O(3) ap atoms found in the [SrO] 0 layers (due to the shorter Al–O(3) ap bond length), the Z * for the remaining ions are closer to the nominal values. It is also worth noting that the magnitude of the anisotropy Δ Z for La and Sr is greater in the η =2 sequence relative to the η =1/3 sequence ( Table 1 ). However, we find Δ Z (La)< 0, similar to η =1/3. Internal electric fields In Fig. 2 , we show the macroscopically averaged [32] , [33] local nuclear ionic potential, excluding contributions of the exchange-correlation and Hartree terms, along the [001] direction obtained from our first-principles calculations for each sequence. The built-in internal electric fields, which are proportional to the gradient in the potential, are the source for the cation-ordering-driven bond-length modulations. The dipolar interactions provide the driving force for the cooperative atomic displacements (as shown in Fig. 1 ), which occur to minimize the interatomic forces for a given η in LaSrAlO 4 . 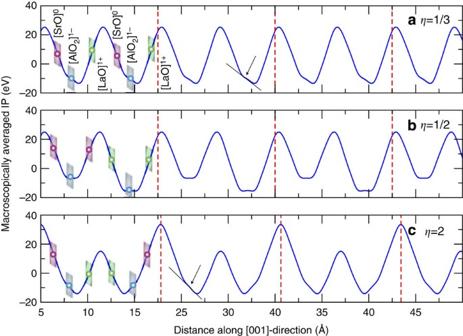Figure 2: Internal electric fields in LaSrAlO4. Macroscopically averaged local ionic potential (IP) along the [001] direction for the (a)η=1/3, (b)η=1/2 and (c)η=2 ordered variants. Charged planes are shown to indicate the minimum in the planar averages for each [LaO]1+(green), [SrO]0(maroon) and [AlO2]1−(blue) layer in the unit cell. Large electric fields (∝slope, arrowed) across the AlO2layers are exceedingly sensitive to the AO monoxide layer sequenceη, for example, 0.92 GV cm−1in (c) relative to 0.41 GV cm−1in (a). Averaging is performed over a window of 2.12 Å, comparable with the interlayer spacings; vertical (red) broken lines represent thec-axis lattice spacing. Figure 2: Internal electric fields in LaSrAlO 4 . Macroscopically averaged local ionic potential (IP) along the [001] direction for the ( a ) η =1/3, ( b ) η =1/2 and ( c ) η =2 ordered variants. Charged planes are shown to indicate the minimum in the planar averages for each [LaO] 1+ (green), [SrO] 0 (maroon) and [AlO 2 ] 1− (blue) layer in the unit cell. Large electric fields ( ∝ slope, arrowed) across the AlO 2 layers are exceedingly sensitive to the AO monoxide layer sequence η , for example, 0.92 GV cm −1 in ( c ) relative to 0.41 GV cm −1 in ( a ). Averaging is performed over a window of 2.12 Å, comparable with the interlayer spacings; vertical (red) broken lines represent the c -axis lattice spacing. Full size image Figure 2a,c clearly depicts the different electric fields that occur across the AlO 2 layers in the η =1/3 and 2 sequences (arrowed). The steeper slope produces a larger asymmetry in the Al–O ap bonds, that is, the magnitude of local electric field across the AlO 2 layers is greater for η =2 than in the η =1/3 sequence. In addition, the field does not cancel in η =1/3 owing to the polar crystal structure. Interestingly, in the η =1/2 sequence the macroscopic average profile of the two perovskite-like blocks, [SrO|AlO 2 |SrO] and [LaO|AlO 2 |LaO] are markedly different ( Fig. 2b ). The local minimum in the macroscopic averages do not coincide in η =1/2 (for example, see filled symbols indicating Al sites), unlike the other two sequences. We anticipate these variations in the internal electric field from cation ordering to alter the positions of the valence and conduction band edges. 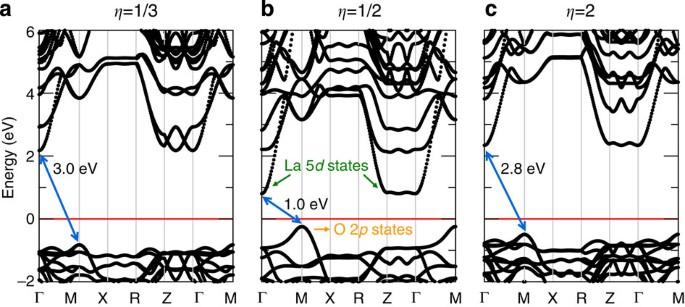Figure 3: Cation ordering driven control over band gaps. Band structures computed at the DFT-PBEsol level for (a)η=1/3, (b)η=1/2 and (c)η=2 LaSrAlO4. All configurations have indirect band gaps, in agreement with experimental optical measurements, which evolves with the [AO] order sequence. The top of the valence bands and bottom of the conduction bands originate from O 2pand La 5dstates, respectively. Electronic structure and band gaps Figure 3 shows the electronic band structures obtained from our DFT-PBEsol simulations for the three cation-ordered sequences. All three configurations are found to be insulating, with the top of the valence band (VB) and bottom of the conduction band (CB) formed mainly from O 2 p and La 5 d states, respectively. Note that the bandwidths of the O 2 p and La 5 d states are also altered as a function of η , but more remarkably, the magnitude of the indirect band gap ( E g , indicated by the blue arrows) is significantly affected by the AO layering sequence. Figure 3: Cation ordering driven control over band gaps. Band structures computed at the DFT-PBEsol level for ( a ) η =1/3, ( b ) η =1/2 and ( c ) η =2 LaSrAlO 4 . All configurations have indirect band gaps, in agreement with experimental optical measurements, which evolves with the [AO] order sequence. The top of the valence bands and bottom of the conduction bands originate from O 2 p and La 5 d states, respectively. Full size image The polar η =1/3 LaSrAlO 4 structure has the largest E g (3.0 eV), followed by the η =2 sequence, which is slightly reduced (2.8 eV). Moreover, the η =1/2 structure with two distinct A- and B-site sublattices has a significantly reduced E g of 1 eV. Note that the inclusion of the La 4 f -states in the pseudopotentials increased the E g of η =1/2 by 0.5 eV, but has a negligible effect on the electronic gaps of η =1/3 and 2 sequences. For η =1/2 LaSrAlO 4 , we find two important changes to the band edges that are notably absent in both η =1/3 and 2 sequences. Figure 3b shows a shift in the band edges and an enhanced dispersion of both the O 2 p states from Γ–M–X, originating from the O(4) eq atoms in the [SrO|AlO 2 |SrO] block in the VB, and the La 5 d states at the bottom of the CB. The combination of these two effects, which are less pronounced in η =1/3 and 2, leads to the massive 2 eV band gap reduction. For comparison, we also report the E g values obtained using an all-electron DFT scheme in Table 2 (see the row labelled Wien2k and the Methods section for details). Although the band gap values of the η =2 and η =1/3 configurations using the full potential method remain essentially unaltered relative to the ultrasoft pseudopotential values (see Table 2 ), the inclusion of the La 4 f states increases the band gap by 0.6 eV in η =1/2. This finding is consistent with results using pseudopotentials that explicitly treat the 4 f states described above. Table 2 Electronic band gaps for LaSrAlO 4 . Full size table Our calculations with the HSE06 functional, which includes a fractional contribution of exact-Fock exchange, and with the Green’s function G 0 W 0 method are known to more accurately reproduce band gaps [34] , [35] also find a similar 2.3 eV reduction for the η =1/2; albeit, as expected, the absolute value of the gap differs between methods ( Table 2 ). The direct Γ→Γ band gaps also show similar behaviour, with that the η =1/2 sequence considerably smaller than that of the η =1/3 and 2 sequences. Origin of gap variation To identify the atomic features responsible for the band gap reduction, we probe the sensitivity of the electronic structure to various lattice distortions appearing in the equilibrium η =1/3, 1/2 and 2 structures. We performed a set of computations starting with the experimental structure of the η =0 LaSrAlO 4 solid solution, where the La- and Sr cations are randomly distributed. The η =0 LaSrAlO 4 belongs to I 4/ mmm space group and its lattice constants a and c are 3.754 and 12.64 Å, respectively. With the η =0 structure, we ordered La and Sr on the A-sites corresponding to the η =1/3, 1/2 and 2 sequences. We next performed self-consistent DFT calculations using ultrasoft pseudopotentials at the PBEsol level of theory, where we neither relaxed the internal coordinates nor the unit cell geometry and calculated the electronic band gap. In this way, we are able to isolate the change in the electronic structure independent of the induced lattice and bond distortions to identify the [LaO] 1+ and [SrO] 0 ordering effect on the band gap. We found that the E g of the η =1/3 and 2 sequences reduced from 3.0 and 2.8 eV, respectively in the ground state (see Table 2 ) to values of 2.77 and 0.16 eV, respectively. In contrast, the η =1/2 sequence became metallic. These calculations when compared with the results obtained from allowing differential ionic relaxations due to the chemical ordering reveal two key effects: (i) the cation ordering drives large band gap variations to such an extent that the η =1/2 sequence becomes metallic and (ii) the critical role of lattice relaxations, that is, variation in the bond lengths (strains) and angles, in response to the cation ordering sequences restores the gap. Our findings highlight the important interplay of electrostatics and local bond strain by [LaO] 1+ and [SrO] 0 ordering to tune the electronic properties of LaSrAlO 4 . The cation order drives a reduction in the E g from the large electric fields (as shown in Fig. 2 ), whereas the screening provided by differential atomic relaxations [36] reduces these field strengths and maintains the insulating behaviour of LaSrAlO 4 . As the variation in the fields for each sequence is different (due to different η values), we arrive at the variation in the E g ( Table 2 ). Furthermore, we also explored the sensitivity of the conduction band edge, (that is, La 5 d states) for the η =1/2 sequence with the smallest E g . We cooperatively displaced the two O ap atoms in the [LaO|AlO 2 |LaO] block, such that P 4/ mmm symmetry is preserved. Supplementary Fig. 5 shows that as the two Al–O ap bond lengths decrease (increase) relative to the ground state configuration, the energy difference between the minimum in the macroscopically averaged local ionic potential between the two perovskite-like blocks increases (decreases). This bond contraction (elongation) results in an increase (decrease) of the indirect band gap ( Supplementary Fig. 5b–d .) As the induced Al–O displacements are produced by the buckling of the LaO monoxide layers in response to the electrostatic effect, our computational exercises conclusively show that the E g changes arises directly from the ordering of [LaO] 1+ and [SrO] 0 monoxide layers in the [001] direction—the cation-ordering-driven bond length modulations provide a direct route to tune band structure using internal electric fields without elemental substitution. Using this principal finding of massive variations in the E g trend without any changes to the stoichiometry through AO monoxide layering induced internal fields, we establish cation ordering as a novel means for electronic structure engineering in materials with well-defined two-dimensional planes. As transition metal oxides exhibit many functional properties, including anisotropic transport, strong electron-lattice coupling (superconductivity and magnetoresistance), relative ease of ion-exchange and intercalation, low thermal conductivity and ferroelectricity (to name a few), this understanding could lead to layered oxides as a platform for multilfunctional and adaptive electronic materials. To realize our theoretical predictions, we suggest thin film growth methods like oxide molecular beam epitaxy (MBE) to be well-suited for experimentally achieving the proposed cation ordering variants [37] , [38] , [39] . Recently, A-site cation ordered LaSrNiO 4 and LaSrMnO 4 RP oxides were experimentally grown with precise atomic control using oxide-MBE techniques [40] , [41] . Leveraging, this approach with misfit strain from epitaxial growth or by tuning the magnitude of the cation-ordering-driven bond length modulations via large A-site valence differences offers a potentially transformative paradigm to rationally design band gaps, absorption and emission edges, or transport properties for photo- and electrocatalysis, where such layered Ruddlesden-Popper and Dion-Jacobson phases are already finding use, yet remains far from ideal. Electronic structure calculations Density functional theory calculations were performed within the generalized gradient approximation (GGA) PBEsol exchange—correlation functional [42] as implemented in the plane-wave pseudopotential code, Quantum ESPRESSO (QE) [43] . In calculations involving QE, the core and valence electrons were treated with ultrasoft pseudopotentials [44] with the inclusion of nonlinear core corrections with a planewave basis (60 Ry cutoff). See Supplementary Note 1 and Supplementary Table 1 for additional calculation details. The following valence electronic configurations were used for our Troullier-Martin [45] pseudopotentials, La: 5 s 2 5 p 6 5 d 1 6 s 2 ; Sr: 4 s 2 4 p 6 5 s 2 ; Al: 3 s 2 3 p 1 ; and O: 2 s 2 2 p 4 . The Brillouin zone integration was performed over a 8 × 8 × 5 Monkhorst-Pack k -point mesh [46] centred at Γ. The atomic positions and the cell volume were relaxed until the Hellmann-Feynman forces and stress tensor <2 meV Å −1 and 0.1 kbar, respectively, were achieved. Lattice dynamical calculations were performed using PHONOPY [47] on a 2 × 2 × 2 supercell with forces obtained from self-consistent total energy calculations using the finite displacement method (see Supplementary Note 2 ). The electric polarization (Δ P ) for the polar LaSrAlO 4 variant is calculated using the Berry phase method [48] . The Born effective-charge tensors ( Z *), which characterize the influence of long-range Coulombic interactions, were calculated using the density functional perturbation theory (DFPT) for the equilibrium structures [49] . We also used the all-electron code Wien2k [50] to validate the suitability of our pseudopotentials for accurately describing the electronic band structure. Wien2k calculations were also performed within the PBEsol exchange-correlation functional. The muffin-tin sphere radii were chosen as follows; La: 2.2, Sr: 2.0, Al: 1.7, O: 1.6 a.u. and we used a plane-wave cutoff of RK MAX =7. The Brillouin zone integration was performed over a 14 × 14 × 4 Monkhorst-Pack k -point mesh [46] centred at Γ. We relaxed the lattice using MSR1a for optimization of positions [51] . Note that the relaxed lattice and internal coordinates from Wiek2k agreed well with the Quantum ESPRESSO simulations. Given the inherent limitation in the DFT exchange-correlation functionals in accurately predicting band gaps, we also used the hybrid exchange-correlation functional HSEsol [52] , and a beyond-DFT ( G 0 W 0 ) method as implemented in the BerkeleyGW [53] , [54] , [55] code to substantiate the band gap variations observed with changes in η . Normconserving pseudopotentials constructed using the OPIUM pseudopotential package ( http://opium.sourceforge.net/ ) were used for the HSEsol and G 0 W 0 calculations. DFT calculations were performed on a 8 × 8 × 5 mesh to obtain well-converged single-electron wave functions using the GGA-PBEsol functional as a starting guess for calculating the quasiparticle energies and wavefunctions within the G 0 W 0 method. The process of computing the quasiparticle energies requires two steps: first, calculation of the static or frequency-dependent polarizabilities ( χ ) and dielectric functions within the random phase approximation (RPA). The generalized plasmon-pole model is used to extend the dielectric function to finite frequency. We used a dielectric cutoff energy of 50 Ry to solve for χ, from which the RPA dielectric matrix is calculated. Second, calculation of the screened Coulomb interaction, W , and the one-particle Green’s function, G , from the inverse dielectric matrix (obtained from Step 1) and DFT eigenfunctions, respectively. These quantities are then used to evaluate the self-energy operator (Σ) and obtain the quasiparticle energies. We used screened coulomb and bare coulomb cutoff values of 10 and 25 Ry, respectively. Additional details on the methodology can be found in the ref. 55 . For η =1/3 and 2 sequences, the complex flavour of the BerkeleyGW code was used. In contrast, we used the real flavour for the η =1/2 sequence. In Supplementary Table 3 , the convergence of the indirect band gap ( E g ) as a function of number of conduction or empty bands is given. How to cite this article: Balachandran, P. V. et al. Massive band gap variation in layered oxides through cation ordering. Nat. Commun. 6:6191 doi: 10.1038/ncomms7191 (2015).